Long-term nitrogen deposition depletes grassland seed banks Nitrogen (N) pollution is a global threat to the biodiversity of many plant communities, but its impacts on grassland soil seed banks are unknown. Here we show that size and richness of an acid grassland seed bank is strongly reduced after 13 years of simulated N deposition. Soils receiving 140 kg N ha −1 per year show a decline in total seed abundance, seed species richness, and the abundance of forbs, sedges and grasses. These results reveal larger effects of N pollution on seed banks than on aboveground vegetation as cover and flowering is not significantly altered for most species. Further, the seed bank shows no recovery 4 years after the cessation of N deposition. These results provide insights into the severe negative effects of N pollution on plant communities that threaten the stability of populations, community persistence and the potential for ecosystems to recover following anthropogenic disturbance or climate change. Atmospheric nitrogen (N) deposition is among the top three threats to global biodiversity [1] . It is estimated that by 2050 global N deposition will be almost twice as high as at the beginning of the 1990s (ref. 2 ), threatening many ecosystems worldwide [3] . Anthropogenic activities have caused an increase in atmospheric N deposition, which in turn has altered the global N cycle radically, threatening the biodiversity of terrestrial and marine ecosystems [4] . In terrestrial ecosystems, several effects of N deposition on aboveground plant communities have been identified, including changes in plant cover, abundance, species composition and richness [4] , [5] , [6] , a decline in resistance to pathogens and pests [4] , [5] , an increase in susceptibility to drought and frost [4] , [5] and a decrease in the stability of biomass production (by the effects of N eutrophication) [6] . The impact of N deposition on soil seed banks is a major concern since they contribute to the maintenance of plant species diversity [7] , buffer small, isolated populations against local extinction [8] , and are key determinants of ecosystem resistance and resilience [9] . Despite widespread evidence of impacts of N pollution on floristic diversity and plant community structure [4] , [5] , studies on soil seed banks are scarce [10] , [11] , [12] , [13] and most are limited to short-term effects. For example, a 3-year study of N addition in a desert community found no change in the density or species richness of the seed bank [11] , while another 1-year study found that N addition increased seedling emergence [12] . One long-term study of N addition showed changes in seed bank composition in a tundra plant community [13] . However, N pollution impacts on grassland seed banks are unknown. In principle N addition could increase seed bank density if the increases in inputs (seed production) dominate, or decrease seed bank density if seed production is reduced, losses from the seed bank are increased or seed bank formation is restricted by the build-up of excessive litter layers [14] . Quantifying the long-term impact of N addition on seed banks is therefore a key missing link in our understanding of ecosystem responses to N pollution, with important implications for grassland conservation and restoration. Here we show the effects of atmospheric N deposition on the soil seed bank in acid grassland plots in the UK that have been exposed to simulated N deposition since 1995, and also in plots allowed to recover (following cessation of treatments) since 2005. The Wardlow site is both one of the earliest and longest running N deposition experiments in the world, simulating atmospheric N deposition on grassland ecosystems [5] . Seed bank analysis was further supported by an evaluation of the vegetative cover and flowering. We demonstrate that N pollution has large and previously unsuspected negative effects on the soil seed bank beneath one of the most widespread and plant-species rich types of acidic grassland in Europe. Specifically, 13 years of simulated N deposition reduced the species richness and abundance of the seed bank, with negative impacts on all the three functional groups: forbs, sedges and grasses. In addition, the seed bank showed no sign of recovery >4 years after cessation of N deposition, even though flowering recovered. These results indicate that N pollution has larger effects on grassland seed banks than on vegetation, providing new insights into the mechanisms of biodiversity loss by this globally intensifying pollutant. Effects on seed bank size and richness We found that total abundance of the seed bank was reduced by 61% and 34% in soils receiving 140 (140N) and 35 (35N) kg N ha −1 per year, respectively ( Fig. 1a ). Moreover, there was a 41% and 29% reduction in species richness in the high and low nitrogen-addition treatments ( Fig. 1b ), an effect not recorded in the aboveground vegetation [5] . Although seed bank composition was changed significantly by N deposition, the correlation between N treatment and seed bank composition was weak ( Supplementary Fig. 1 ). 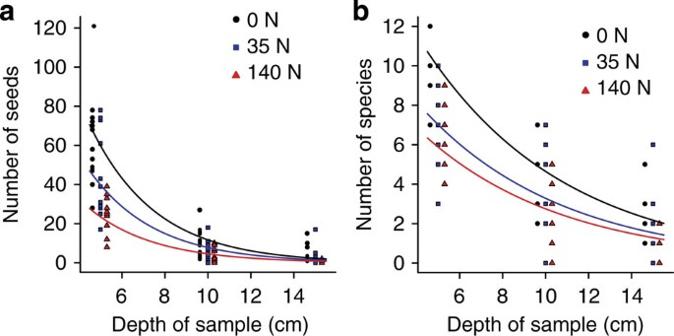Figure 1: Effect of nitrogen deposition on the soil seed banks of an acid grassland after 13.5 years of experimental N addition at Wardlow Hay Cop. (a) Number of seeds. (b) Number of species. Both 35N and 140N deposition rates reduced the total seed abundance significantly (GLMM; −0.41±0.14;z=−2.9,P<0.01 and −0.94±0.15;z=−6.4,P<0.00001, respectively). Moreover, species richness decreased under 35 N (GLMM; −0.35±0.11;z=−3.2,P<0.01) and 140N (GLMM; −0.52±0.12;z=−4.5,P<0.00001). A significant decrease in the (a) number of seeds (GLMM; −0.33±0.01;z=−34.7,P<0.00001) and (b) the number of species (GLMM; −0.15±0.01;z=−11.6,P<0.00001) was recorded with the increasing soil sample depth across all the treatments. The figure shows the scatter plots with the fitted curves. Each point is the number obtained by adding the values of four soil samples in every individual plot (n=108). Figure 1: Effect of nitrogen deposition on the soil seed banks of an acid grassland after 13.5 years of experimental N addition at Wardlow Hay Cop. ( a ) Number of seeds. ( b ) Number of species. Both 35N and 140N deposition rates reduced the total seed abundance significantly (GLMM; −0.41±0.14; z =−2.9, P <0.01 and −0.94±0.15; z =−6.4, P <0.00001, respectively). Moreover, species richness decreased under 35 N (GLMM; −0.35±0.11; z =−3.2, P <0.01) and 140N (GLMM; −0.52±0.12; z =−4.5, P <0.00001). A significant decrease in the ( a ) number of seeds (GLMM; −0.33±0.01; z =−34.7, P <0.00001) and ( b ) the number of species (GLMM; −0.15±0.01; z =−11.6, P <0.00001) was recorded with the increasing soil sample depth across all the treatments. The figure shows the scatter plots with the fitted curves. Each point is the number obtained by adding the values of four soil samples in every individual plot ( n =108). Full size image Effects on functional groups and the most abundant species For all the three main functional groups, there were significant reductions in seed bank abundance of forbs (73%), sedges (56%) and grasses (56%) in soils receiving 140N. However, in soils receiving 35N only the abundance of grasses was reduced significantly (34%) ( Fig. 2 ). Among the eight most abundant species in the seed bank, four species showed no significant reduction in the number of seeds (generalized linear mixed model (GLMM); P >0.1 in all the cases) by either 35N or 140N deposition rates ( Agrostis capillaris × stolonifera , Carex pilulifera , Holcus lanatus and Poa pratensis ). The abundance of three species was reduced significantly by the 140N rate, Agrostis vinealis by 61% (GLMM; estimate±s.e. of the estimate of the fixed effect parameter in the model=−0.92±0.39; z -test=−2.4, P =0.02), Galium saxatile by 70% (GLMM; −1.22±0.42; z =−2.9, P <0.01) and Potentilla erecta by 76% (GLMM; −1.43±0.34; z =−4.3, P <0.0001), while abundance of A. capillaris was reduced significantly by both 35N (56%, GLMM; −0.82±0.33; z =−2.5, P =0.01) and 140N deposition rates (70%, GLMM; −1.19±0.33; z =−3.6, P <0.001). 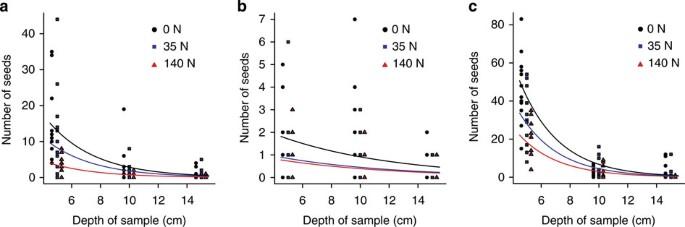Figure 2: Effect of nitrogen deposition on the number of seeds of the three main functional groups in the soil seed bank after 13.5 years of N addition at Wardlow Hay Cop. (a) Forbs. (b) Sedges. (c) Grasses. The 140N deposition rate reduced the number of seeds of forbs significantly (GLMM; −1.33±0.3;z=−4.5,P<0.00001) and sedges (GLMM; −0.85±0.39;z=−2.2,P=0.03) while 35N did not have a significant effect on both the number of seeds of forbs (GLMM; −0.45±0.28;z=−1.6,P=0.1) and sedges (GLMM; −0.71±0.38;z=−1.9,P=0.06). Both 35N and 140N treatments reduced the number of seeds of grasses significantly (GLMM; −0.41±0.18; z=−2.3,P=0.02 and −0.83±0.18;z=−4.5,P<0.00001, respectively). A significant decrease in the number of seeds of (a) forbs (GLMM; −0.3±0.02;z=−16.8,P<0.00001), (b) sedges (GLMM; −0.12±0.03;z=−4.3,P<0.0001) and (c) grasses (GLMM; −0.37±0.01;z=−29.6,P<0.00001) was recorded with increasing soil sample depth across all treatments. The figure shows the scatter plots with the curves. Each point is the number obtained by adding the values of four soil samples in every individual plot (n=108). Figure 2: Effect of nitrogen deposition on the number of seeds of the three main functional groups in the soil seed bank after 13.5 years of N addition at Wardlow Hay Cop. ( a ) Forbs. ( b ) Sedges. ( c ) Grasses. The 140N deposition rate reduced the number of seeds of forbs significantly (GLMM; −1.33±0.3; z =−4.5, P <0.00001) and sedges (GLMM; −0.85±0.39; z =−2.2, P =0.03) while 35N did not have a significant effect on both the number of seeds of forbs (GLMM; −0.45±0.28; z =−1.6, P =0.1) and sedges (GLMM; −0.71±0.38; z =−1.9, P =0.06). Both 35N and 140N treatments reduced the number of seeds of grasses significantly (GLMM; −0.41±0.18; z=−2.3, P =0.02 and −0.83±0.18; z =−4.5, P <0.00001, respectively). A significant decrease in the number of seeds of ( a ) forbs (GLMM; −0.3±0.02; z =−16.8, P <0.00001), ( b ) sedges (GLMM; −0.12±0.03; z =−4.3, P <0.0001) and ( c ) grasses (GLMM; −0.37±0.01; z =−29.6, P <0.00001) was recorded with increasing soil sample depth across all treatments. The figure shows the scatter plots with the curves. Each point is the number obtained by adding the values of four soil samples in every individual plot ( n =108). Full size image Effect of the aboveground vegetation response on seed banks The impacts of N deposition on the seed bank do not simply reflect the response of the aboveground vegetation; in fact we found reduced similarity between the seed bank and the aboveground plant community in plots receiving 140N treatment ( Supplementary Fig. 2 ). Moreover, cover of only one species, P. erecta was reduced significantly by 140N deposition (generalized linear model (GLM); F=9.8; df=2,33; P <0.001; t =−4.4, P< 0.001) but not by 35N (GLM; t =−1.9, P =0.06), while flowering in the same species was reduced at both 35N and 140N deposition rates (GLM; F=14.5; df=2,33; P< 0.0001; t =−3.5, P =0.01 and t =−6.1, P = < 0.00001, respectively). Cover and flowering of the other species was not affected significantly by 35N or 140N treatment (GLM; P >0.1 in all the cases). Although exotic species in the seed bank can increase after N deposition [11] , we did not record any weeds or invasive species in the soil, which is consistent with the aboveground vegetation responses [5] . Seed bank recovery Four years after experimental N deposition ceased, there was no significant recovery in any of the seed bank characteristics (total abundance (GLMM; 0.12±0.12; z =0.99, P =0.32), richness (GLMM; −0.01±0.09; z =−0.093, P =0.93), or the abundance of forbs (GLMM; 0.22±0.23; z =0.97, P =0.33), sedges (GLMM; 0.09±0.3; z=0.31, P =0.76), grasses (GLMM; 0.02±0.15; z =0.12, P =0.91) or the abundance of individual species ( A. vinealis (GLMM; −0.22±0.31; z =−0.7, P =0.5), G. saxatile (GLMM; 0.28±0.33; z =0.84, P =0.4), P. erecta (GLMM; 0.24±0.24; z =1.0, P =0.31) and A. capillaris (GLMM; −0.26±−0.26; z =−1.0, P =0.31)). This is despite the flowering of P . erecta recovering following cessation of both 35N and 140N treatments (GLM; F=6; df=2,30; P< 0.01; t =2.6, P =0.01 and t =3.3, P< 0.01, respectively). Over a large geographical scale, evidence indicates that chronic nitrogen deposition has decreased plant species richness in acid grasslands in Europe [15] . At local scale, a 2004 UK-wide survey in areas of contrasting N deposition revealed a major impact of N deposition on the species diversity of acid Festuca – Agrostis pasture, a very abundant type of upland grassland throughout northern Europe [16] . We have now demonstrated a large impact of experimental N deposition on the size and diversity of the soil seed bank beneath the same grassland type. This impact is of major concern owing to the role of seed banks in population recovery and vegetation management. The mechanisms underpinning these changes are unknown, but several possibilities seem likely ( Fig. 3 ). First, it is well known that N-containing compounds including nitrate, nitrite and ammonium stimulate seed germination in many species, and therefore N pollutants might diminish the seed bank by promoting seed germination [10] , [12] , [17] , [18] , [19] . N deposition also acidifies soils [20] , which has complex effects on seed germination, but may promote germination in some species, either directly [21] or indirectly (for example, by the effects of increasing toxic metal levels [22] , [23] and microbial growth and composition [24] ). The attack by pathogenic microorganisms is a major source of seed mortality in soil, and it may be that one effect of N deposition is to promote microbial seed pathogenesis [25] . Certainly N deposition can increase the susceptibility of established plants to pathogens [5] . Moreover, a higher N content of the seed coat in relation to C (carbon) content may provide an improved nutritional resource for decomposer microorganisms [25] , [26] . It may also be that the negative impacts of N deposition on flowering that have been recorded in some communities, lead to a reduction in seed production [5] . Finally, high N addition can increase litter build-up, which may act as a barrier to the entry of seeds to the seed bank [14] . Our results do not allow us to attribute the decline in the seed bank to a single cause, but in the case of P. erecta , which showed both a decline in the seed bank and significant reductions in cover (under 140N deposition) and flowering (under both 35N and 140N depositions), reduction in seed production is likely to have been important. In contrast, graminoids increased in vegetation cover [5] , suggesting that the decline in grass and sedge seed banks is more related to the losses of seeds from the soil than to reduced seed inputs. Overall, changes in the seed bank were more severe than changes in the aboveground plant communities, suggesting that the main effect of N deposition on the seed bank operates via belowground processes. 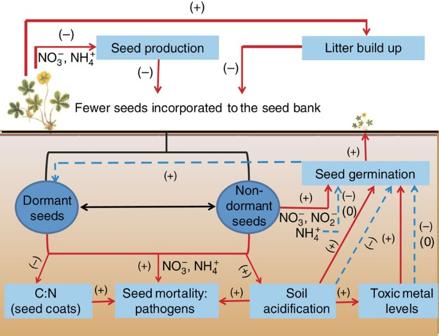Figure 3: Simplified scheme of the potential causes of soil seed bank depletion by N pollution. The unidirectional red solid arrows represent processes affecting seed bank size. The positive, negative or neutral direction of the impacts is indicated by (+), (−) and (0), respectively. Blue dashed lines show alternative mechanisms of seed bank depletion based on the species-specific effects of N pollution on seeds (not discussed above). N-containing compounds, soil acidification and phytotoxic metals may have a negative21,22,43,44or neutral22,44effect on germination, and therefore can increase the size of the seed bank through increased seed dormancy. Greater seed availability to microorganisms can then increase seed mortality with time. Figure 3: Simplified scheme of the potential causes of soil seed bank depletion by N pollution. The unidirectional red solid arrows represent processes affecting seed bank size. The positive, negative or neutral direction of the impacts is indicated by (+), (−) and (0), respectively. Blue dashed lines show alternative mechanisms of seed bank depletion based on the species-specific effects of N pollution on seeds (not discussed above). N-containing compounds, soil acidification and phytotoxic metals may have a negative [21] , [22] , [43] , [44] or neutral [22] , [44] effect on germination, and therefore can increase the size of the seed bank through increased seed dormancy. Greater seed availability to microorganisms can then increase seed mortality with time. Full size image Impoverishment of grassland floras by N deposition is clearly widespread [5] , [15] , [27] , with no reason to assume that depletion of grassland seed banks is not equally common, with potentially large effects on diversity, composition and functioning of grassland ecosystems. Such impoverishment threatens to increase the local extinction risk by reducing the capacity of the plant populations to recover from disturbance [9] . Loss of the seed bank also degrades a reservoir of genetic diversity [28] and therefore the ability of the community to respond to habitat alteration [29] and environmental change [30] . Finally, seed bank loss not only jeopardizes the natural ability of grasslands to recover from hazards such as fire, drought or overgrazing, but also limits the usefulness of seed banks as a source of plant material for the use in ecological restoration programmes. Particularly worrying is the failure of grassland seed banks to show any evidence of recovery after the N deposition ceases. This occurred despite flowering of some species (for example, P . erecta ) recovering following the cessation of treatments and total potassium-chloride extractable mineral nitrogen in the top soil rapidly falling back to control values even in the 140N plots [31] . The lack of seed bank response indicates that the recovery process is slow, although recovery may be possible in the long term. Our results suggest that future studies should measure the time lags between the above and belowground processes and between the vegetation and seed banks. Moreover, seed bank conservation and recovery should be an integral part of grassland restoration programmes. Study site On the basis of previous studies [20] , [32] , an acidic grassland was chosen to investigate the effects of long-term atmospheric nitrogen deposition on seed banks. The grassland is located on the south-east facing slope (5–10°) of a conical hill at Wardlow Hay Cop, in the South Pennines, in Cressbrook Dale National Nature Reserve within the Peak District National Park, UK (53°15’44N, 1°44’02W), and 370 m.a.s.l ( [20] ). During the past century, Wardlow Hay Cop has received one of the highest rates of N pollutant deposition in the United Kingdom [20] , [32] . Therefore, although the highest application treatment (140N) exceeds the current deposition rates reported for the UK, this treatment was chosen because the South Pennines region received cumulative N deposition in the 20th century amounting to 2,200–3,200 kg N ha −1 , equating to between 22–33 kg ha −1 per year [33] . Our treatment application rates thus ranged from rates similar to historical deposition rates (35 kg N ha −1 per year above ambient values in 1995) to the 140N treatment that equates to application rates used in agricultural practices [32] . Since the main form of N deposition in upland areas is wet deposition, the treatments have been applied monthly in 2 l of distilled water, per plot per application, as a mist by using a backpack sprayer [20] . The acidic grassland is situated over a Carboniferous limestone bedrock, which has been covered with paleo-argillic brown earth from the Nordrach series [34] that reaches 70-cm deep [35] . Owing to the thickness of the soil and the excess of precipitation in relation to evapotranspiration, the bedrock does not have an effect on the soil pH in the surface layers, therefore the soil is extremely acidic in the surface layer where pH ranges from 3.5 to 4.0 and has been acidified by acid rain [20] . The organic-matter-rich surface soil horizons are 12–15-cm deep, dark brown, humus-rich, stoneless, silty loam [20] , with ~40% organic matter content [36] . The subsurface mineral horizons [20] reach the bedrock and are stoneless, silty clay loam with clay and sesquioxide translocation [34] , [37] . The vegetation of the area is classified as a Festuca–Agrostis–Galium grassland of NVC U4e (ref. 38 ). The community is part of the Derbyshire Dales National Nature Reserve currently managed by Natural England. The long-term nitrogen and phosphorus deposition plots Plots (3 × 3 m) have been receiving N treatments of 35 (35N) or 140 (140N) kg N ha −1 per year of NH 4 NO 3 in factorial combination with 35 kg P ha −1 per year of NaH 2 PO 4 , or no added P, since September 1995; controls receive distilled water only [20] , [32] . Since January 2005, half of each plot has continued to receive one of the treatments while the other half (‘recovery plots’) has not. The treatments were applied in a fully randomized block design replicated three times (3N × 2P × 3 blocks) [32] . Each replicate block consisted of six 3 × 3 m plots, split in half (3 × 1.5 m) to establish the recovery treatments. Seed bank sampling and characterization Inside each 3 × 1.5 m plot, soil samples were removed in March–April 2009, before spring germination and seed set and after natural winter stratification. To minimize the disturbance to the plots, four soil cores, 4.5 cm in diameter, were taken from the centre of each plot (72.5 cm to the right and left of the edge of the plot). The first core was taken at 60 cm from the top of the plot, the second one in the middle (120 cm from the top), the third in the middle (180 cm from the top) and the last one at the bottom (60 cm from the bottom of the plot). The samples were subdivided at 5-cm depth intervals (0–5 cm, 5.1–10 cm and 10.1–15 cm) for processing and analysis. The experiment also included a phosphorus addition treatment; however, as this did not alter any of the seed bank characteristics (GLMM; P >0.1) it was dropped from the analysis. The total number of soil samples per plot was 12, 144 per block and 432 per all the three blocks. The total volume of soil samples in every plot was 1178, cm 3 . Characterization of seed banks took place following the recommendations of Thompson et al . [39] The vegetative parts of plants were removed from soil samples [39] . Then, the samples were sieved (2.8 mm, 2 mm and 710 μm) and spread in germination trays in a layer of 1–3 mm on top of compost (Levington Professional Growing Medium-M3 High Nutrient: peat based, standard pH (5.5–6) and low conductivity (450–550 μS). In addition, 100 germination trays were filled with compost only to test for background seed contamination. All trays were randomly distributed in the greenhouse (Unigro Grodome growth chambers at The Arthur Willis Environment Centre in The University of Sheffield) and maintained under 16-h photoperiod with a temperature of 15 °C (night) and 25 °C (day). Light was supplied by high-pressure sodium bulbs, which provided an irradiance of 183 μmol m −2 s −1 at bench height. The light and temperature were controlled by an automatic environment system (Unigro Building Management System). All trays were watered daily from below with tap water. Seedling emergence was recorded weekly from April 2009 to January 2010. Seedlings were removed soon after being identified to species. Flowering characterization The number of flowers ( P. erecta ) or inflorescences ( A. capillaris, A. vinealis, H. lanatus, P. pratensis, C. pilulifera and G. saxatile ) per 3 × 1.5 m plot were counted during summer 2011. Counts of all grass and forb species took place between 12th and 16th July, at peak flower abundance, determined from frequent visual inspections of the site during known flowering periods, and before the main period of sheep and cattle grazing at the site (late July to mid September). Inflorescences of the spring flowering sedge, C. pilulifera , were counted on 9th June. Strings were used to divide each of the plots into eighteen, 0.5 × 0.5 m squares to facilitate accurate counting. Inflorescences touching the outer strings were considered to be within the plot only if originating from an individual rooted within the plot. Vegetation percentage cover characterization The percentage cover of all species was recorded in ten, 0.5 × 0.5 m quadrats placed contiguously, 0.25 m from the outer margins of each 1.5 × 3 m plot, during the period 27th July–3rd August 2011. Estimates were made to the nearest 5%, with the exception of species comprising <5% cover, which were recorded as 1, 2 and 3%. Separation of the grass species A. capillaris and A. vinealis could not be reliably undertaken within an appropriate timescale and was not attempted. Values from the ten quadrats were averaged to produce an estimated cover for each plot. Statistical analysis The seed bank response variables were number of species, total number of seeds, number of seeds of each functional group (forbs, grasses and sedges) and number of seeds of the eight most abundant species. GLMMs were fitted using the R-package lme4 (refs 40 , 41 ) with treatment (nitrogen and/or the recovery treatments) and depth of the sample as the fixed effects and plot as a random effect with the Poisson error distributions. Flowering data were square-root transformed and analysed using a linear model (Gaussian errors, identity link). Mean percentage cover data for G. saxatile , P. erecta and P. pratensis were arcsine transformed and analysed using a linear model (Gaussian errors, identity link). For Agrostis spp. and H. lanatus cover was analysed using quasi-Poisson models and a log link function. Too few individuals of C. pilulifera were recorded aboveground and so no statistical analysis was conducted for this species. All statistical analyses and figures were performed in R [40] . To visualize the changes in the seed bank across treatments, composition data were ordinated by NMDS (non-metric multidimensional scaling), using a Bray–Curtis distance measure. Analyses were performed with the meta-MDS function in the vegan package in R [40] , [42] . The default square root and double-Wisconsin transformations were disabled and the effect of data transformations was tested manually; square-root transformation did not substantially alter NMDS stress values or species and site scores, therefore analyses are based on untransformed values. The aboveground plant community and seed bank were compared using Bray–Curtis distance. Seed bank data were converted to relative abundance and vegetation survey data to relative cover to avoid differences in sampling scales. How to cite this article : Basto, S. et al . Long-term nitrogen deposition depletes grassland seed banks. Nat. Commun. 6:6185 doi: 10.1038/ncomms7185 (2015).